Cephalopod-inspired design of electro-mechano-chemically responsive elastomers for on-demand fluorescent patterning Cephalopods can display dazzling patterns of colours by selectively contracting muscles to reversibly activate chromatophores – pigment-containing cells under their skins. Inspired by this novel colouring strategy found in nature, we design an electro-mechano-chemically responsive elastomer system that can exhibit a wide variety of fluorescent patterns under the control of electric fields. We covalently couple a stretchable elastomer with mechanochromic molecules, which emit strong fluorescent signals if sufficiently deformed. We then use electric fields to induce various patterns of large deformation on the elastomer surface, which displays versatile fluorescent patterns including lines, circles and letters on demand. Theoretical models are further constructed to predict the electrically induced fluorescent patterns and to guide the design of this class of elastomers and devices. The material and method open promising avenues for creating flexible devices in soft/wet environments that combine deformation, colorimetric and fluorescent response with topological and chemical changes in response to a single remote signal. Soft material systems that are flexible, remotely controllable and capable of emitting fluorescence and light are playing critical roles in nontraditional displays for applications as diverse as stretchable electronics, foldable lighting devices, flexible and biocompatible luminescent recourses for clinical therapy, and dynamic camouflage [1] , [2] , [3] , [4] , [5] , [6] , [7] , [8] , [9] , [10] . To design these responsive soft material systems, various strategies have been exploited, such as embedding rigid light-emitting diodes into elastomeric substrates [3] , [4] , [5] , [6] , [7] , employing stretchable electro-luminescent polymers [1] , [8] , [9] , [11] and designing microfluidic networks filled with controlled pigment fluids [10] , [12] , [13] , [14] , [15] . On the other hand, nature offers a drastically different strategy that enables soft skins of animals to spontaneously display versatile colours and fluorescence [10] , [16] , [17] . For example, cephalopods (including cuttlefish, octopuses and squids) [16] , [17] , [18] , [19] can display dazzling patterns of colours for signalling or active camouflage in response to environmental stimuli. The colouration generally relies on skin chromatophores composed of pigment-containing sacs that are attached to multiple radial muscles [16] , [20] ( Fig. 1a,b ). By contracting and releasing the muscles, the corresponding pigment sacs can expand and shrink their areas, reversibly producing various colourful patterns such as spots, trenches and bands within short-time scales (for example, within seconds) [16] , [20] . The selection of chromatophores to be activated is usually controlled by the cephalopod’s nervous system in response to environmental stimuli. This natural display strategy, if successfully implemented in engineering devices, would greatly benefit and advance various fields such as flexible electronics, photonics, dynamic camouflage and biomedical luminescent devices [1] , [2] , [3] , [4] , [5] , [6] , [7] , [8] , [9] , [10] . Despite its potential, both the development of new materials for chromatophores and the design of remote-control mechanisms for chromatophore devices are challenging tasks in materials science and technology [17] , [19] . 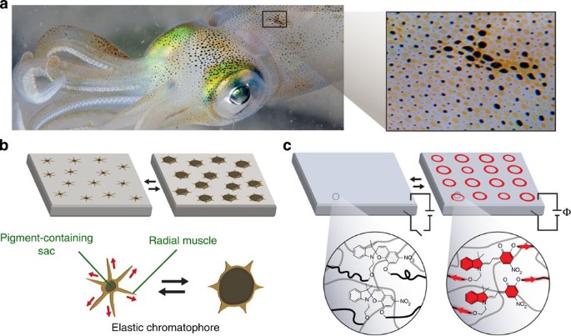Figure 1: Bioinspired design strategy for on-demand fluorescent patterning. (a,b) Schematic of the colouration mechanism employed by cephalopods. Skin chromatophores of a squid (photograph courtesy of Klaus Stiefel) are composed of pigment-containing sacs that are attached to multiple radial muscles. By contracting and releasing the muscles, the corresponding pigment sacs expand and shrink their surface area coverage. (c) Schematics of the mechanism for on-demand fluorescent patterning controlled by applied voltage. The applied voltages induce various patterns of large deformation on the surface of an EMCR elastomer, which subsequently exhibits corresponding fluorescent patterns. Figure 1: Bioinspired design strategy for on-demand fluorescent patterning. ( a , b ) Schematic of the colouration mechanism employed by cephalopods. Skin chromatophores of a squid (photograph courtesy of Klaus Stiefel) are composed of pigment-containing sacs that are attached to multiple radial muscles. By contracting and releasing the muscles, the corresponding pigment sacs expand and shrink their surface area coverage. ( c ) Schematics of the mechanism for on-demand fluorescent patterning controlled by applied voltage. The applied voltages induce various patterns of large deformation on the surface of an EMCR elastomer, which subsequently exhibits corresponding fluorescent patterns. Full size image Here we report a soft material system that employs an electro-mechano-chemically responsive (EMCR) elastomer as an artificial chromatophore and uses electric fields to trigger self-assembled patterns of colour and fluorescence on demand ( Fig. 1c ). To design the EMCR elastomer, we covalently couple a stretchable elastomer with spiropyran mechanophores [21] that change colour and emit strong fluorescent signals when subjected to mechanical stresses. We then integrate the EMCR elastomer into a display panel that can be remotely controlled. Voltages applied to the display panel induce various patterns of large deformation on the surface of the EMCR elastomer, and the induced stresses in turn lead to a versatile range of fluorescent patterns including lines, circles and letters on demand [22] , [23] , [24] , [25] . The activation of EMCR elastomer and fluorescent patterning are reversible and repeatable over multiple cycles, in contrast to the irreversible plastic deformation or fracture required for activating most existing mechanoresponsive polymers [21] , [26] , [27] , [28] , [29] , [30] , [31] , [32] , [33] , [34] . By integrating diverse fluorescent patterns, remote control by voltages and reversibility over multiple cycles, the new cephalopod-inspired EMCR elastomers open promising avenues for creating flexible devices that combine deformation, colorimetric and fluorescent response with topological and chemical changes that might eventually be useful in a variety of applications in soft/wet environments, including flexible displays [3] , [4] , [5] , [6] , [7] , [8] , [9] , [11] , optoelectronics [1] , [8] , [9] , biomedical luminescent devices [2] , [4] and dynamic camouflage coatings [10] , [17] . Fabrication and characterization of the EMCR elastomer The EMCR elastomer is fabricated by covalently coupling the mechanophore spiropyran [21] into the cross-linked network of the silicone elastomer Sylgard 184 (see Methods and Supplementary Fig. 1a for details of the fabrication procedure). The spiropyran is bis-functionalized with terminal alkenes and incorporated into the Sylgard network through platinum cure hydrosilylation reaction [35] ( Supplementary Fig. 1 ). The Sylgard elastomer under sufficiently large deformation (for example, >125% strain) transfers the macroscopic force to the spiropyran groups and triggers a 6-π electrocyclic ring-opening reaction that reversibly transforms a near-colourless spiropyran to a highly coloured merocyanine that is also strongly fluorescent [21] , [26] , [30] ( Supplementary Figs 1b and 2 ). The deformation of the elastomer can also be induced by applying electric fields [36] , [37] , [38] , a concept we exploit here to enable reversible electro-mechano-chemical response in elastomeric display devices. We first characterize the colour change and fluorescence of the EMCR elastomer under mechanical deformation. As the elastomer film is uniaxially stretched, the initially pale yellow elastomer turns dark blue [35] ( Fig. 2a,b ). In addition, we acquire fluorescent images of the deformed EMCR elastomers by exciting them with ~545 nm green light and collecting emission between 590 and 650 nm (see Methods). The EMCR elastomers exhibit different fluorescent intensities under different strains ( Fig. 2d ). We quantify the fluorescence intensity of the elastomer as a function of the uniaxial strain, which is defined as ε =( L – L 0 )/ L 0 , where L 0 and L are the side lengths of the elastomer film in the undeformed and deformed states, respectively (see Methods on the procedure to quantify the fluorescent density). From Fig. 2e , it can be seen that the fluorescence intensity maintains at a relatively low level when the strain in the elastomer is low (that is, <125% strain). As the elastomer is deformed above 125% strain, the fluorescence intensity begins to increase monotonically with increasing strain as more and more spiropyrans in the elastomer are activated. This stagnant-increasing trend is observed in EMCR elastomer films with various spiropyran concentrations from 0.05% wt to 0.5% wt, and the fluorescence intensity is proportional to spiropyran content ( Fig. 2e ). 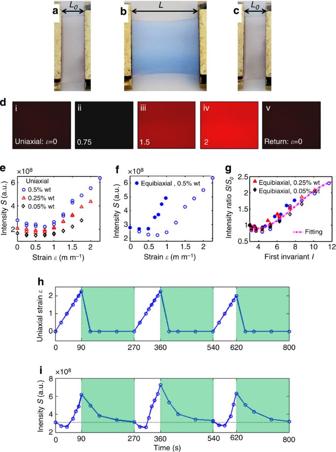Figure 2: Characterization of colour change and fluorescence of EMCR elastomer films. (a,b) Colour change of an EMCR Sylgard film under a uniaxial strain of 200%. (c) The relaxed EMCR film after being exposed to green light (~545 nm) for 3 min. (d) Fluorescent microscope images of the film under various uniaxial strains. (e) Fluorescent intensitiesSplotted as functions of applied uniaxial strain and spiropyran concentration. (f) Fluorescent intensities of the EMCR films with 0.5% wt spiropyran as functions of uniaxial strain and equibiaxial strain. (g) Normalized fluorescence intensity as a function of the first invariant of deformed EMCR films with various spiropyran concentrations and strains. (h,i) Cyclic uniaxial strain applied to an EMCR film and the corresponding fluorescence intensity. The green shadow domains indicate that the EMCR film is under green light (~545 nm) for 3 min. Figure 2: Characterization of colour change and fluorescence of EMCR elastomer films. ( a , b ) Colour change of an EMCR Sylgard film under a uniaxial strain of 200%. ( c ) The relaxed EMCR film after being exposed to green light (~545 nm) for 3 min. ( d ) Fluorescent microscope images of the film under various uniaxial strains. ( e ) Fluorescent intensities S plotted as functions of applied uniaxial strain and spiropyran concentration. ( f ) Fluorescent intensities of the EMCR films with 0.5% wt spiropyran as functions of uniaxial strain and equibiaxial strain. ( g ) Normalized fluorescence intensity as a function of the first invariant of deformed EMCR films with various spiropyran concentrations and strains. ( h , i ) Cyclic uniaxial strain applied to an EMCR film and the corresponding fluorescence intensity. The green shadow domains indicate that the EMCR film is under green light (~545 nm) for 3 min. Full size image Besides uniaxial deformation, the EMCR elastomer film can also be stretched biaxially. To obtain a general relation between deformation and fluorescence in the elastomer, we plot the fluorescence intensity of the elastomer under equibiaxial strains in Fig. 2f (see Supplementary Fig. 3 for the deformation schematics). As seen by comparing Fig. 2e,f , the same strain gives greater activation under biaxial deformation than uniaxial deformation. As the mechanophores are activated within stretched polymer chains, we choose the commonly used first invariant of the Cauchy-Green deformation tensor I =(1+ ε 1 ) 2 +(1+ ε 2 ) 2 +(1+ ε 3 ) 2 to characterize the degree of stretching in polymer chains, where ε 1 , ε 2 and ε 3 are principal strains in the elastomer [39] , [40] . Therefore, for an elastomer film under uniaxial strain ε , the first invariant can be calculated as I =(1+ ε ) 2 +(1+ ε ) −2 +1; and for a film under equibiaixal strain ε , the first invariant is I =2(1+ ε ) 2 +(1+ ε ) −4 ( Supplementary Fig. 3 ). By plotting the normalized fluorescence intensity as functions of I , the curves for elastomers with different spiropyran concentrations and under both uniaxial and biaxial loadings all collapse on one master curve ( Fig. 2g ), where S 0 and S are fluorescent intensities of the EMCR elastomer in the undeformed and deformed states, respectively. The master curve can be fitted to a polynomial function f ( I )=−0.004 I 3 +0.098 I 2 −0.557 I +1.816. In this way, the fluorescence intensity in the elastomer film for a given deformation can be predicted using equation (1). In contrast to most mechanophore-bearing polymers, which are usually plastically deformed or fractured during the first activation [21] , [26] , [27] , [28] , [29] , [30] , [31] , [32] , [33] , [34] , the Sylgard-based EMCR elastomers are reversible and repeatable [33] over multiple loading–unloading cycles [35] ( Fig. 2h,i ), and it instantaneously recovers its undeformed state from very large deformation (for example, 200% strain) once unloaded. A colourless and non-fluorescent film can be quickly recovered by illuminating the relaxed EMCR elastomer with green light (wavelength ~545 nm) to accelerate the ring-closing reaction [35] ( Fig. 2c , Supplementary Fig. 1b ). Figure 2h shows that the fluorescent intensity of the relaxed elastomer decreases by 80% under 1 min of exposure to green light, and fully returns to the level of the undeformed state within 3 min. On-demand fluorescent patterning with the EMCR elastomer On-demand fluorescent patterns are achieved by integrating the EMCR elastomer into a display panel under the control of applied electric fields. 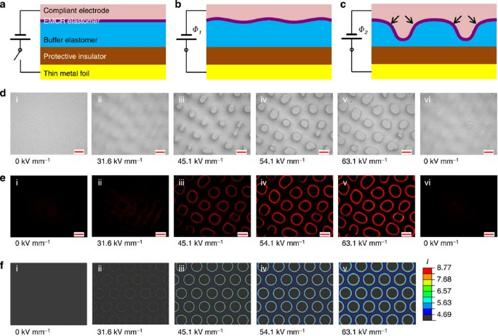Figure 3: Electro-mechanical activation of EMCR elastomer films. Schematic illustrations of (a) the experimental setup, (b) wrinkle initiation and (c) crater formation. The arrows incindicate the locations of large deformation in the EMCR film. The fluorescence intensity of the EMCR film is first equilibrated to a force-free photostationary state by being exposed to green light for 3 min, and then activated with ramping electric field. (dI–VI) Optical microscope and (eI–VI) fluorescent microscope images of the EMCR film under varied electric fields. Image VI ofeis the EMCR film illuminated by the green light for 3 min. The thicknesses of EMCR elastomer, buffer elastomer and protective insulator are ~21, ~106 and 125 μm, respectively. The applied voltages through (dI–dV) are 0, 3, 10, 12 and 14 kV, respectively. The scale bars indandedenote 250 μm. (fI–V) Finite-element calculations of the first invariant in the EMCR film under increasing electric field. Figure 3 demonstrates the design and working mechanism of the display panel. The EMCR elastomer film is bonded to an underlying buffer elastomer whose shear modulus is lower than that of the EMCR elastomer. To protect the whole system from electric breakdown, the elastomer bilayer is laminated onto a protective insulator with much higher electric strength and modulus than the elastomers. An electric field is applied to this laminate through an external direct-current voltage that is connected to a thin gold layer coated on the bottom surface of the protective insulator, and a compliant electrode is used to cover the top surface of the elastomer bilayer. The compliant electrode, NaCl solution [37] , [38] , is transparent and can deform conformally with the elastomer bilayer surface. Figure 3: Electro-mechanical activation of EMCR elastomer films. Schematic illustrations of ( a ) the experimental setup, ( b ) wrinkle initiation and ( c ) crater formation. The arrows in c indicate the locations of large deformation in the EMCR film. The fluorescence intensity of the EMCR film is first equilibrated to a force-free photostationary state by being exposed to green light for 3 min, and then activated with ramping electric field. ( d I–VI) Optical microscope and ( e I–VI) fluorescent microscope images of the EMCR film under varied electric fields. Image VI of e is the EMCR film illuminated by the green light for 3 min. The thicknesses of EMCR elastomer, buffer elastomer and protective insulator are ~21, ~106 and 125 μm, respectively. The applied voltages through ( d I– d V) are 0, 3, 10, 12 and 14 kV, respectively. The scale bars in d and e denote 250 μm. ( f I–V) Finite-element calculations of the first invariant in the EMCR film under increasing electric field. Full size image Once an applied electric field reaches a critical value, the initially flat surface of the EMCR elastomer becomes unstable and forms a pattern of wrinkles ( Fig. 3b,dII , and Supplementary Movie 1 ). The pattern of wrinkles resembles those observed in bilayer systems induced by thermal expansion [41] , [42] , swelling [43] , [44] and ultraviolet or ion irradiation treatment [45] , [46] . As the applied electric field further rises, the valleys of the wrinkles are pinched down, forming a pattern of craters ( Fig. 3c , Fig. 3dIII–dV , and Supplementary Movie 1 ). Once the electric field is withdrawn, the instability pattern spontaneously disappears upon elastic recovery and the surface of the EMCR elastomer returns to the flat state ( Fig. 3dVI and Supplementary Movie 1 ). As the deformation of the EMCR film is relatively low in the flat and wrinkled states, the fluorescence intensity remains at background levels at the corresponding electric fields ( Fig. 3eII and Supplementary Movie 2 ). At higher electric fields, however, the formation of craters involves large deformations ( I>6 ) in the EMCR film around the crater edges, and the mechanophores are activated and emit strong fluorescent signals ( Fig. 3c , Fig. 3eIII–eV and Supplementary Movie 2 ). As shown in Fig 3e , fluorescent patterns of rings are formed around the craters, and the fluorescent intensity becomes stronger with increasing electric field. As a control experiment, the fluorescence of a Sylgard elastomer film incorporating a bis-functionalized and mechanically inactive spiropyran (that is, molecular elongation does not lead to ring-opening) remains low under the same applied electric fields ( Supplementary Movies 3 and 4 ), confirming that electro-mechano-chemical coupling to stress-bearing polymer subchains is necessary to activate the mechanophores. Nearly, full reversibility and repeatability of the whole pattern are seen over multiple on/off cycles ( Supplementary Movie 2 ). When the applied electric field is ramped up to 63.1 kV mm −1 , the observed maximum fluorescence intensity in the pattern gradually increases to 1.8 times of the initial intensity of the film at 0 kV mm −1 ( Fig. 4a,b ). Thereafter, the applied electric field is withdrawn and the EMCR elastomer film is continuously irradiated with green light. Consequently, the maximum fluorescence intensity decreases dramatically to ~1.15 times of the initial intensity in 30 s, and returns to the initial intensity within 3 min ( Fig. 4a,b ). Remarkably, the reversible patterning can be repeated over 100 cycles ( Fig. 4a,b ). 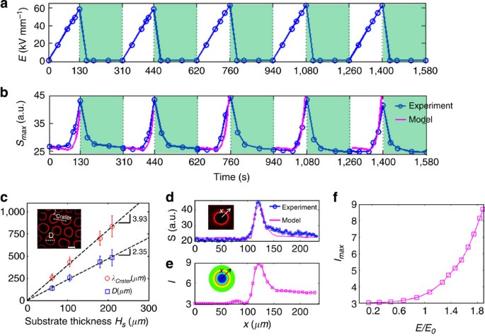Figure 4: Fluorescence intensity and feature size of the field-induced fluorescent patterns. (a) Cyclic electric fields applied to the EMCR film and (b) the corresponding fluorescence intensity. The green shadow domains indicate that the EMCR film is under green light (~545 nm) for 3 min. (c) Crater wavelengths and internal diameters of the fluorescent rings as a function of the thickness of the buffer substrate. (d) Fluorescence intensity and (e) calculated first invariant of the EMCR film along a radial path of the fluorescent ring. (f) The maximum first invariant in EMCR film as a function of applied electric field. The critical electric field for wrinkling instability isE0=33.5 kV mm−1. Figure 4: Fluorescence intensity and feature size of the field-induced fluorescent patterns. ( a ) Cyclic electric fields applied to the EMCR film and ( b ) the corresponding fluorescence intensity. The green shadow domains indicate that the EMCR film is under green light (~545 nm) for 3 min. ( c ) Crater wavelengths and internal diameters of the fluorescent rings as a function of the thickness of the buffer substrate. ( d ) Fluorescence intensity and ( e ) calculated first invariant of the EMCR film along a radial path of the fluorescent ring. ( f ) The maximum first invariant in EMCR film as a function of applied electric field. The critical electric field for wrinkling instability is E 0 =33.5 kV mm −1 . Full size image Next, we analyse the physics of the electrically induced pattern formation and provide a predictive model for the deformation and fluorescent emission of the EMCR elastomer film under applied electric fields. Assuming that the EMCR and buffer elastomers follow the ideal dielectric law [47] , the Gibbs free energy of the system (that is, elastomer bilayer and the voltage) can be expressed as where V f and V s denote representative volumes of the EMCR film and the buffer substrate; W Mf and W Ms the strain energy density of the EMCR film and the buffer substrate; κ the permittivity of the EMCR film and the buffer substrate; E the electric field vector in the domain. We further define the uniform electric field in flat regions of the EMCR film as the applied electric field E . The three terms in equation (2) denote the electrostatic potential energy, the strain energy of the EMCR film and the buffer substrate, respectively. The surface energy has negligible effect in the current study [38] , [48] . The electrically induced pattern formation is driven by the decrease of electrostatic potential energy and resisted by the increase of strain energy. By dimensional argument, the critical electric fields for the onset of wrinkling instability in the elastomer bilayer can be expressed as [48] where Ψ is a dimensionless function of modulus ratio μ f / μ s and thickness ratio H f / H s , and μ f , μ s and H f , H s are the shear modulus and thickness of the EMCR film and the buffer substrate, respectively. Similarly, by dimensional argument, the wavelength of the wrinkle at the onset can be expressed as [48] where Ω is another dimensionless function of μ f / μ s and H f / H s . We use the linear stability analysis to calculate Ψ and Ω (see Supplementary Methods , Supplementary Fig. 5 ). We further analyse the evolution of caters that emerge after the wrinkling instability. To characterize the wavelength of the craters, we experimentally vary the thickness of the buffer substrate, finding that the crater wavelength closely follows λ crater ≈3.93 H s , on the same order as λ 0 in equation (4) ( Fig. 4d ). The internal diameter of the fluorescent rings follows a similar law as D ≈2.35 H s , also on the same order as λ 0 ( Fig. 4d ). The crater depth increases significantly with the rise of applied electric field, causing large deformation in the EMCR film around the edge of the crater ( Fig. 3c ). To further calculate the magnitude of electric fields that induce craters with different depths, we compare the Gibbs free energy of the cratered and flat states calculated numerically with equation (2) as a function of the applied electric field [47] (see Supplementary Methods and Supplementary Fig. 6 ). Applying the Maxwell stability criterion [47] , the depth of the resulting craters will vary with the magnitude of applied electric field, stretching the EMCR film to different degree ( Supplementary Fig. 6b ). As shown in Fig. 4e , the calculated first invariant I in the EMCR film under applied electric fields features a sharp peak at the edge of the crater, which corresponds to the location of maximum fluorescence intensity in Fig. 4d . Recalling the relationship between I and fluorescence intensity from equation (1), we can predict the fluorescence intensity along a radial path of the crater under an applied field, for example, 63.1 kV mm −1 . As seen in Fig. 4d , the theoretical prediction agrees well with the experimental observation. In addition, the maximum first invariant I in the EMCR film increases monotonically with the applied electric field ( Fig. 4f and Supplementary Fig. 6e ) as which can be fitted to a polynomial function g ( E / E 0 )≈0.41( E / E 0 ) 4 +0.12( E / E 0 ) 2 +3. Combining equation (1) and equation (5), we obtain an empirical formula for the maximum fluorescence intensity in the EMCR film as a function of the applied electric field. Figure 4b demonstrates good agreement between the observed and calculated intensity. To further validate the hexagonally distributed fluorescent-ring patterns in Fig. 3e , we perform finite-element simulations of the patterns of hexagonally distributed craters in Supplementary Fig. 7 . The calculated first invariants in the patterns in Fig. 3f qualitatively match the experimentally observed fluorescent rings in Fig. 3e . The display devices reported here are inspired by the capability of dynamic colour changes in cephalopod skins, and apply a similar hierarchy of signal-to-strain-to-colour to an EMCR elastomer that can reversibly and repeatedly fluoresce in response to electromechanical loadings. Here the mechanisms at play occur on the higher resolution length scale of cross-links within a polymer network, and we capitalize on this resolution in voltage-controlled display panels that can reversibly display fluorescent patterns on demand. In addition to the hexagonal patterns of fluorescent rings demonstrated in Fig. 3e, a number of other patterns can also be achieved. For example, we can align the fluorescent rings by pre-deforming the EMCR film. Before bonding the EMCR elastomer film on the buffer substrate, we uniaxially pre-stretch the film by a ratio of λ p ( Fig. 5a ). This pre-stretch induces a tensile stress that partially offsets the electrically induced stress in the EMCR film along the pre-stretch direction [37] ( Fig. 5a ). The electrically induced wrinkle therefore tends to align along the pre-stretch direction because of lower compressive stress in that direction ( Supplementary Fig. 8 ). Subsequently, the crater patterns will develop along the aligned valleys of the wrinkles under higher applied electric fields. For instance, when λ p is small (for example, 1.16), craters are shown to align uniformly along the valleys of aligned wrinkles ( Fig. 5a ), and the corresponding fluorescent rings are also aligned along the pre-stretch direction ( Fig. 5b ). When λ p is large (for example, 1.82), however, the valleys of the aligned wrinkles tend to become deeper, resulting in a pattern of trenches ( Fig. 5d ). The trench edges feature localized large deformation and thus exhibit strong fluorescent lines ( Fig. 5e ). The fluorescent intensities along characteristic paths are also well predicted by finite-element calculations ( Fig. 5b,c,e and f ). 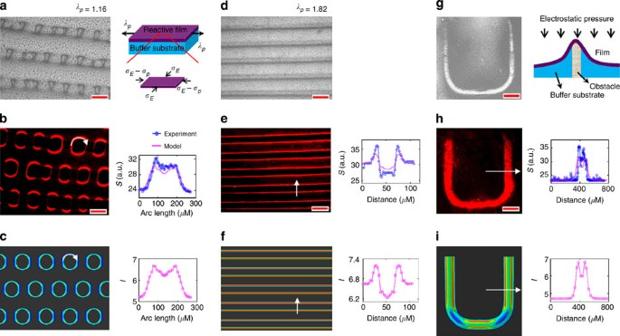Figure 5: On-demand fluorescent patterns formed by EMCR elastomers under electric fields. (a) Optical microscope image, (b) fluorescent microscope image and (c) calculated first invariant in the EMCR film with aligned crater patterns under applied field of 68.5 kV mm−1(applied voltage is 15 kV). The inset inaillustrates the stress state of the pre-stretched EMCR film under an electric field. The inset inbshows the fluorescence intensity along a semi-circumference path of a fluorescent ring (indicated as a cured arrow). The inset ofcshows the calculated first invariant along the path. (d) Optical microscope image, (e) fluorescent microscope image and (f) calculated first invariant of trenches formed in the pre-stretched EMCR film under applied field of 59.1 kV mm−1(applied voltage is 12.8 kV). The insets ofeandfshow the fluorescence intensity and calculated first invariant along indicated paths, respectively. Ina,b,dande, the thicknesses of EMCR elastomer and buffer elastomer are ~21 and ~106 μm, respectively. (g) Optical microscope image, (h) fluorescent image and (i) calculated first invariant of a ‘U’ pattern in the EMCR film bonded on a buffer substrate embedded with a rigid object. The inset ingillustrates the mechanism of the pattern formation. The insets ofhandishow the fluorescence intensity and calculated first invariant along indicated paths, respectively. Ingandh, the thicknesses of EMCR elastomer and buffer elastomer are ~21 and ~100 μm, respectively; the applied voltage is 17 kV. The scale bars ina,b,d,e,gandhdenote 250 μm. Figure 5: On-demand fluorescent patterns formed by EMCR elastomers under electric fields. ( a ) Optical microscope image, ( b ) fluorescent microscope image and ( c ) calculated first invariant in the EMCR film with aligned crater patterns under applied field of 68.5 kV mm −1 (applied voltage is 15 kV). The inset in a illustrates the stress state of the pre-stretched EMCR film under an electric field. The inset in b shows the fluorescence intensity along a semi-circumference path of a fluorescent ring (indicated as a cured arrow). The inset of c shows the calculated first invariant along the path. ( d ) Optical microscope image, ( e ) fluorescent microscope image and ( f ) calculated first invariant of trenches formed in the pre-stretched EMCR film under applied field of 59.1 kV mm −1 (applied voltage is 12.8 kV). The insets of e and f show the fluorescence intensity and calculated first invariant along indicated paths, respectively. In a , b , d and e , the thicknesses of EMCR elastomer and buffer elastomer are ~21 and ~106 μm, respectively. ( g ) Optical microscope image, ( h ) fluorescent image and ( i ) calculated first invariant of a ‘U’ pattern in the EMCR film bonded on a buffer substrate embedded with a rigid object. The inset in g illustrates the mechanism of the pattern formation. The insets of h and i show the fluorescence intensity and calculated first invariant along indicated paths, respectively. In g and h , the thicknesses of EMCR elastomer and buffer elastomer are ~21 and ~100 μm, respectively; the applied voltage is 17 kV. The scale bars in a , b , d , e , g and h denote 250 μm. Full size image In addition, the fluorescent pattern can be tailored by pre-modulating the substrate geometry. We embed in the buffer substrate an object with designed geometry but much higher modulus than the EMCR film and the buffer substrate ( Fig. 5g , Supplementary Fig. 9 ). Under applied electric field, the EMCR film is forced to pinch into the buffer substrate but blocked by the embedded rigid object, thus forming a protruded pattern that replicates the geometry of the object. As shown in Fig. 5g , the electrically induced topography reproduces the shape of the embedded object, a letter ‘U’. Strong fluorescence is also observed to follow the geometry of the letter ‘U’, because the EMCR film is significantly deformed around the rigid object ( Fig. 5h ). Further numerical simulations predict the fluorescence intensity and can be used to guide the design of future patterns ( Fig. 5i and Supplementary Fig. 10 ). In terms of practical applications, we point out that the actuation electric fields reported here are ~50 kV mm −1 and the laminate thickness is ~200 μm, so the actuation voltages in the current experiments are on the order of 10 kV. Voltages of this magnitude do present a challenge for breakdown, but it is not prohibitive; similar electric fields and voltages are employed, for example, in dielectric-polymer actuators that have been used in practical applications such as haptic keyboards and tactile covers for portable electronic devices [49] , [50] . In addition, the breakdown electric field of the protective insulating layer in the laminate is ~160 kV mm −1 – much higher than the applied fields here, suggesting that even this first-generation system can work reliably over time without electrical breakdown [37] , [38] . Looking ahead, opportunities for reducing the required voltage include decreasing the thickness of the laminate. Guidance along those lines is found in our finite-element model in Supplementary Fig. 11 , which shows that a substrate-film thickness ratio H s / H f ≥1 is needed to ensure significant deformation in the EMCR elastomer under electric fields (that is, the maximum first invariant in the EMCR elastomer must be larger than 6). Therefore, in order to reduce the actuation voltage, one can reduce the overall thickness of the laminate as long as the substrate-film thickness ratio is kept above 1. There is an obvious trade off here that would need to be optimized in the context of a given application, because a thinner EMCR elastomer will give lower intensity of fluorescent emission. Finally, the components of the EMCR elastomer might be improved, either by activating brighter fluorophores or employing better polymers. Along the latter lines, we note that ionic polymers that give large deformation under low-electric fields (for example, ~10 V mm −1 ) have recently been reported [51] . The design principles presented in this paper should help guide developments in all of the above areas. In summary, we demonstrate a bioinspired soft material system for generating voltage-controlled on-demand fluorescent patterns that can be modulated to exhibit manifold geometries. As a model for new types of displays, this design paradigm should be easily translatable to optoelectronic devices comprising various luminescent polymers and activated by various stimuli [1] , [2] , [3] , [4] , [5] , [6] , [7] , [8] , [9] , [10] , [11] , [52] , [53] , [54] . The dimension of the current display panel is 2 cm by 2 cm and the feature size of the florescent patterns is ~100 μm. The size of the display can be potentially scaled up by using larger pieces of elastomer laminates covered by compliant and transparent electrodes, as demonstrated in previous studies on patterning of larger-area elastomer surfaces with electric fields [37] , [55] . As the feature size of the patterns scales with the elastomer buffer’s thickness ( Fig. 4c ), the resolution of the display may be further enhanced (if desired) by decreasing the thickness of the buffer elastomer. In the context of mechanoresponsive polymers, these systems represent a first generation of mechanochemical devices, in which localized covalent chemical changes (here, the conversion of spiropyran to merocyanine) and their association function can be turned on and off repeatedly in response to an external signal remotely controlled. Numerous mechanophores with chemical functionality including catalysis [56] , [57] and small molecule release [33] , [35] have been reported, and mechanochemical coupling offers the potential to add chemical response to existing soft device functionality. To that end, the development of material platforms that can trigger covalent mechanochemistry while recovering their initial shape [33] , [35] motivates the need for new mechanophores that, like the materials, are reversibly and repeatably activated. Preparation of EMCR elastomers The EMCR Sylgard film is prepared as described previously [35] . The active [35] and control [21] spiropyrans are synthesized as previously reported and bis-functionalized with terminal alkenes. The functionalized spiropyrans are dissolved in xylenes (Sigma-Aldrich) and mixed with the base and curing agent (10:1 by weight) of Sylgard 184 (Ellsworth Adhesives). The spiropyran is crosslinked into Sylgard network by a platinum-catalysed hydrosilylation reaction, the same curing chemistry as that between vinyl- and hydrosilane functionalities in the initial Sylgard networks. The concentration of spiropyran is varied from 0.05% wt to 0.5% wt for the active spiropyran and 0.5% wt for the control. The solution is spin-coated onto a BoPET film (McMaster-Carr), followed by polymerization in a vacuum oven at 65 °C for 12 h. The film thickness, controlled by the spin speed, is varied from 15 to 300 μm. The modulus of the EMCR elastomer is measured by the uniaxial tension test (Micro-strain analyzer, TA Instruments) and fitted to the Arruda-Boyce model [39] ( Supplementary Fig. 4 ). Characterization of the fluorescence intensity The EMCR Sylgard film (~300 μm) is first illuminated by a green light (wavelength ~545 nm, 3 min) to obtain a photostationary equilibrium, and then stretched by a uniaxial stretcher (S. T. Japan-USA) or a home-made biaxial stretcher with a slow strain rate (0.025 s −1 ). Fluorescent images are obtained on a Nikon Eclipse LV100 microscope outfitted with a Nikon Intensilight C-HGFI mercury lamp as the illumination source. The objective is × 5 MUE41050 LU Plan Fluor. The fluorescent filter is TRITC Hy Q Cube (EX530-560, DM570, BA590–650). Images are acquired on a Nikon DS-Qi1Mc camera and saved as a 16-bit greyscale tiff images (width 2.22 mm and 1.78 mm height). The fluorescence intensity is calculated by integrating the grey intensity in the acquired image. Fluorescent images in Figs 2d , 3e , 5b, 5e-5h , have been coloured using the LUT command (Red Hot) of Image J. Electro-activation of EMCR elastomers Figure 2a illustrates the experimental setup for electro-activation of EMCR Sylgard films. A direct current voltage is applied between two electrodes using a high-voltage supply (Matsusada). The elastomer bilayer (EMCR elastomer and buffer substrate) is bonded on a protective insulating polymer (Kapton, 125 μm, shear modulus 0.8 Gpa, McMaster-Carr). The soft buffer elastomer is a Sylgard film with a base-to-crosslinker ratio of 125:2 by weight, giving a shear modulus ~1.36 kPa. The applied electric field in the EMCR film is calculated by E =Φ/( H f + H s + H r κ / κ r ), where H f , H s and H r are the thickness of the EMCR Sylgard film, buffer substrate and protective insulator, respectively; Φ is the applied voltage; κ =2.65 κ 0 and κ r =3.5 κ 0 are the permittivity of EMCR film and protective insulator, and κ 0 =8.85 × 10 −12 Fm −1 is the permittivity of vacuum. Finite-element calculations To calculate the electric field and the first invariant in the EMCR film in the cratered state, a finite-element software, ABAQUS 6.10.1, is used to calculate the Gibbs free energy of the elastomer-voltage system ( Supplementary Fig. 7 ). The EMCR film and buffer substrate are taken to obey Arruda-Boyce and ideal dielectric laws [36] , [38] ( Supplementary Fig. 4 ). The two-dimensional ( Supplementary Fig. 6 ) and three-dimensional models ( Supplementary Figs 7,8 and 10 ) are discretized by CPE4RH and C3D8R elements. The result accuracy is ascertained through mesh refinement studies. How to cite this article : Wang, Q. et al. Cephalopod-inspired design of electro-mechano-chemically responsive elastomers for on-demand fluorescent patterning. Nat. Commun. 5:4899 doi: 10.1038/ncomms5899 (2014).